The oil palmVIRESCENSgene controls fruit colour and encodes a R2R3-MYB Oil palm, a plantation crop of major economic importance in Southeast Asia, is the predominant source of edible oil worldwide. We report the identification of the VIRESCENS (VIR) gene, which controls fruit exocarp colour and is an indicator of ripeness. VIR is a R2R3-MYB transcription factor with homology to Lilium LhMYB12 and similarity to Arabidopsis PRODUCTION OF ANTHOCYANIN PIGMENT 1 ( PAP1 ). We identify five independent mutant alleles of VIR in over 400 accessions from sub-Saharan Africa that account for the dominant-negative virescens phenotype. Each mutation results in premature termination of the carboxy-terminal domain of VIR, resembling McClintock’s C1-I allele in maize. The abundance of alleles likely reflects cultural practices, by which fruits were venerated for magical and medicinal properties. The identification of VIR will allow selection of the trait at the seed or early-nursery stage, 3-6 years before fruits are produced, greatly advancing introgression into elite breeding material. Commercially grown oil palm ( Elaeis guineensis ) is an outbreeding diploid species (2 n =32) of West African origin [1] , [2] , [3] . We recently reported the genome sequences of E. guineensis and the South American oil palm, E. oleifera [3] , as well as the discovery of the oil palm SHELL gene, a homologue of SEEDSTICK ( STK ), responsible for oil palm fruit forms [4] . We next sought to identify the genetic basis of oil palm fruit colour. Fruit colour is an important trait in terms of fruit harvesting and, therefore, oil yield. The majority of oil palms produce either nigrescens or virescens fruit type [2] . Nigrescens fruits are usually deep violet to black at the apex and yellow at the base when unripe, with minimal change in colour of the apex upon ripening ( Fig. 1a,c ). Virescens fruits are green when unripe, and change to orange when the bunch matures ( Fig. 1b,c ), reflecting degradation of chlorophyll and accumulation of carotenoids [5] . For nigrescens palms, harvesters rely on the presence of detached fruits on the ground to determine that bunches are ripe. However, as virescens fruits undergo a more profound colour change upon ripening, it is easier to identify ripe bunches, particularly in tall palms where they can be obscured by fronds, thus minimizing yield loss due to fallen fruits or harvesting of unripe bunches. Both nigrescens and virescens palms occur in natural groves. Although the virescens trait is dominant, the number of virescens palms found in natural populations is small, with frequencies ranging from below 1% in Nigeria and Angola [2] to up to 50% in one location in Congo [6] . Virescens palms were used in ancient ceremonial rites [7] , explaining their occurrence among wild-type nigrescens palms, and ‘Ojuku’ trees matching the description of virescens palms were reportedly used in tribal sacrificial ceremonies in West Africa [8] , [9] . 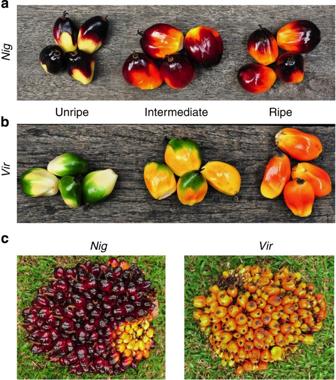Figure 1: Fruit exocarp colour phenotypes. (a) Individual oil palm fruits from anigrescens(Nig) fruit bunch. Unripe fruits are deep-violet to black at the apex (visible in the bunch) and undergo minimal colour change upon ripening. (b) Individual oil palm fruits from avirescens(Vir) fruit bunch. Unripe fruits are green at the apex and change to reddish orange upon ripening. (c) ripenigrescensandvirescensfruit bunches. Figure 1: Fruit exocarp colour phenotypes. ( a ) Individual oil palm fruits from a nigrescens ( Nig ) fruit bunch. Unripe fruits are deep-violet to black at the apex (visible in the bunch) and undergo minimal colour change upon ripening. ( b ) Individual oil palm fruits from a virescens ( Vir ) fruit bunch. Unripe fruits are green at the apex and change to reddish orange upon ripening. ( c ) ripe nigrescens and virescens fruit bunches. Full size image Here, we identify the oil palm VIRESCENS gene and five independent, but remarkably similar mutant alleles of VIR . Phylogenetic analyses and transcriptome studies of virescens and nigrescens fruit suggest that VIR controls oil palm fruit exocarp pigmentation by coordinately regulating expression of genes involved in the anthocyanin biosynthetic pathway. The discovery of alleles responsible for the virescens phenotype, segregating within commercially relevant germplasm collections, has direct applications to the breeding and production practices of the predominant source of edible oil worldwide. Genetic mapping of the VIR locus Oil palm is an outbreeding species, and as such, a high degree of heterozygosity is expected. A population of 240 palms derived from the self-pollination of the tenera palm, T128 (0.151/128 × 0.151/128), from Malaysian Palm Oil Board’s (MPOB) Nigerian germplasm collection [10] , [11] , [12] was used to generate a genetic linkage map [3] , [4] . In addition, a subset of 81 palms from six independent crosses ( Supplementary Table 1 ) was used to confirm marker linkage (Methods). 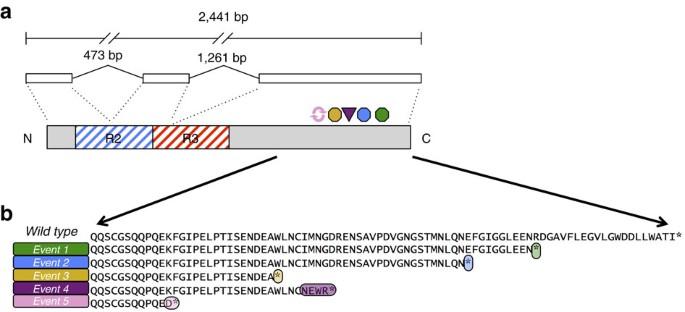Figure 2: Five independentVIRmutations account forvirescensfruit exocarp colour phenotype. (a) Diagram of theVIRgene. The 2.4-kb locus (top line) includes three exons (open boxes) encoding the regions of the R2R3-MYB protein, as indicated by dashed lines. The protein (bottom diagram) includes two helix-loop-helix motifs, R2 and R3. Symbols above the C-terminal domain represent relative positions of the event 1–5 mutations. Symbol colours indicate the specific mutational event as shown in panelb. (b) Protein sequence of the carboxy-terminal region of VIR encoded by wild-type and mutantVIRalleles. Nonsense point mutations (events 1–3), a 2-bp frameshift deletion (event 4) and a rearrangement (event 5) each results in premature termination at the indicated amino-acid position. DNA sequences and details of the event 5 rearrangement are provided inSupplementary Figs 3 and 4. Markers were scored as co-dominant, segregating in a 1:2:1 ratio in most cases, while the virescens phenotype also showed the expected 3:1 segregation ratio in the mapping population ( Supplementary Table 2 , Methods). Three informative restriction-fragment length polymorphism (RFLP) markers were genotyped on the entire mapping population, and 197 SSR loci that were polymorphic in the mapping population were identified. Of 4,451 single-nucleotide polymorphisms (SNPs) screened, 711 were used in map construction. The locus for the virescens gene (VIR) was located on linkage group 1 (chromosome 1), with the RFLP marker MET16 being the most tightly linked ( Supplementary Tables 3 and 4 ; Supplementary Fig. 1 ). Linkage of MET16 to the virescens trait was further tested in the 81 trees, resulting in 95% accuracy for distinguishing between nigrescens and virescens fruit traits ( Supplementary Table 5 ). Markers flanking the VIR candidate locus were mapped by sequence similarity to the E. guineensis ( pisifera ) reference genome assembly [3] and localized to assembly scaffold 7 (p3-sc00007). 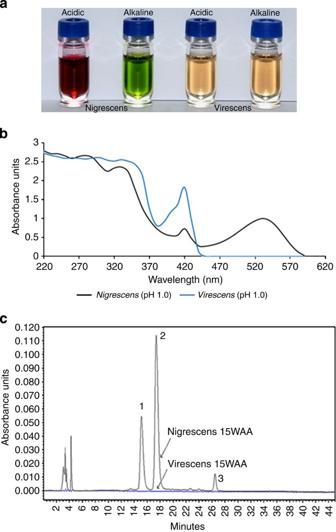Figure 5: Anthocyanin profiles in thevirescensandnigrescensexocarp. (a) Exocarp extracts in acidic and alkaline conditions. Thenigrescensextract was brilliant red in acidic conditions and turned green under alkaline conditions. Thevirescensextract, however, was light orange and did not change under alkaline conditions. (b) Ultraviolet–visible spectrophotometric profile of the extracts at pH 1.0.Nigrescensexhibited a maximum absorbance peak at about 520 nm. This peak was not observed invirescens. Anthocyanins are known to absorb strongly around this wavelength. (c) HPLC profile at 520 nm. Thenigrescensextract had at least three major anthocyanin peaks at 520 nm, which were absent invirescens. A tiling path of bacterial artificial chromosome contigs corresponding to scaffold 7 was selected from a high-information content physical map of pisifera and sequenced. Additional SNP assays were designed from an improved assembly corresponding to scaffold 7 and genotyped (Methods). Markers mapping close to the VIR locus were identified ( Supplementary Fig. 2 ) and markers SNPM02708 and SNPM02400 were positioned on each side of the VIR locus. The interval contained four potential candidate genes that impact fruit pigmentation in other species: a gene with homology to Lilium (lily) LhMYB12 and significant similarity to both Arabidopsis PRODUCTION OF ANTHOCYANIN PIGMENT 1 ( PAP1 ) and AtMYB113 , and three genes with significant similarity to Arabidopsis TRANSPARENT TESTA 12 ( TT12 ), PURPLE ACID PHOSPHATASE 18 ( PAP18 ) or the BHLH gene, ILR3 . VIR mutations responsible for virescens fruit To extend beyond the E. guineensis reference genome sequence, we queried genome sequence assemblies of 12 independent T128 progeny palms (5 nigrescens and 7 virescens ) derived from 20-fold raw sequence coverage (HISEQ 2000) per genome (Methods). Contigs from each assembly were mapped to the scaffolds that had been linked to genetic markers in the virescens genetic interval. In addition, the candidate genes above were each amplified by PCR, including exons and introns, and sequenced ( Supplementary Note 1 ). The entire open-reading frame of the gene homologous to Lilium LhMYB12 and similar to Arabidopsis PAP1 and AtMYB113 was intact in all five nigrescens palms. However, all seven virescens palms were either heterozygous ( n =4) or homozygous ( n =3) for an A-to-T nonsense mutation in exon 3 of the identified candidate VIR gene ( Supplementary Figs 3 and 4 ). The exon 3 mutation results in a predicted truncation of the 21 carboxy-terminal amino acids within the transcriptional activation domain of the R2R3-MYB transcription factor ( Fig. 2 ). Subsequently, the entirety of the gene was amplified and sequenced in 208 trees from the T128 cross (48 nigrescens and 160 virescens ). In all, 158 trees were either heterozygous ( n =99) or homozygous ( n =59) for the nonsense mutation in exon 3, and 50 trees were homozygous wild type, for an overall concordance of this nonsense mutation (event 1) with fruit colour phenotype of 99% ( Table 1 ). It is noted that a 1% discordance rate is well within the norms of phenotyping accuracy of breeding populations [4] . Although SNPs were identified in the other three candidate genes, the polymorphisms observed were not consistent with a functional mechanism affecting fruit colour phenotype of the 12 trees, and independent mutant alleles (see below) were not identified ( Supplementary Note 1 ). Figure 2: Five independent VIR mutations account for virescens fruit exocarp colour phenotype. ( a ) Diagram of the VIR gene. The 2.4-kb locus (top line) includes three exons (open boxes) encoding the regions of the R2R3-MYB protein, as indicated by dashed lines. The protein (bottom diagram) includes two helix-loop-helix motifs, R2 and R3. Symbols above the C-terminal domain represent relative positions of the event 1–5 mutations. Symbol colours indicate the specific mutational event as shown in panel b . ( b ) Protein sequence of the carboxy-terminal region of VIR encoded by wild-type and mutant VIR alleles. Nonsense point mutations (events 1–3), a 2-bp frameshift deletion (event 4) and a rearrangement (event 5) each results in premature termination at the indicated amino-acid position. DNA sequences and details of the event 5 rearrangement are provided in Supplementary Figs 3 and 4 . Full size image Table 1 Summary of VIR genotypes. Full size table To further support the discovery of the VIR gene, we sequenced the entire gene in six independent breeding populations, as well as samples from germplasm collections ( Table 1 ). The breeding populations included 139 trees, where the fruit colour phenotype was known (DT35, DT38, DP454, TT108, MPOB PK575 and a collection of palms from the AVROS background). In addition, 440 trees from Angola, Madagascar, Tanzania, Ghana, Congo, Cameroon and Nigeria were analysed. In the breeding populations, all 52 virescens , but none of the 87 nigrescens trees were found to be either heterozygous or homozygous for the event 1 nonsense mutation in exon 3 ( Table 1 ). However, among the germplasm collections, the event 1 mutation was detected in only 5 of 87 virescens trees, all of which were from either the Ghana or Nigeria collections. Instead, four independent, but closely related mutations were identified in the other germplasm collections from sub-Saharan Africa. First, a G-to-T nonsense mutation (event 2) was detected in exon 3, 30 base pairs (bp) 5′ to event 1 ( Fig. 2 ; Supplementary Figs 3 and 4 ). This mutation results in a predicted truncation of the 31 carboxy-terminal amino acids within the transcriptional activation domain. Event 2 was heterozygous or homozygous in 68 trees from the Angola ( n =45), Tanzania ( n =14), Ghana ( n =4) or Congo ( n =5) collections ( Table 1 ; Fig. 3 ). Next, a G-to-A nonsense mutation (event 3) was detected in exon 3, 113 bp 5′ to event 1 ( Fig. 2 ; Supplementary Figs 3 and 4 ). This mutation results in a predicted truncation of the 59 carboxy-terminal amino acids. The event 3 mutation was heterozygous in 10 trees from Angola ( n =1), Ghana ( n =8) or Congo ( n =1) ( Table 1 ; Fig. 3 ). A fourth mutation (event 4) is a 2-bp deletion beginning 11 bp 3′ to event 3, resulting in translation frameshift at the 55th carboxy-terminal amino acid ( Fig. 2 ; Supplementary Figs 3 and 4 ), and was heterozygous in three trees from Angola and Congo ( Table 1 ; Fig. 3 ). Finally, a heterozygous rearrangement (event 5) resulting in a translational frameshift and premature truncation was detected in three of three virescens trees from Cameroon ( Table 1 ; Figs 2 and 3 ; Supplementary Figs 3 and 4 ). The mutation is a 195-bp deletion with a 21-bp duplication, which results in the truncation of 75 carboxy-terminal amino acids and a single amino-acid conversion before reading a new stop codon. Considering all five single-gene mutations, the concordance between genotype and fruit colour is 99.2% ( Table 1 ). The identification of five independent genetic mutations, each resulting in remarkably similar premature truncation, provides strong evidence for the identification of the VIR gene. C-terminal truncations of related genes in the R2R3-Myb family, most notably the maize C1 gene, have similarly dominant-negative allelic forms [13] . 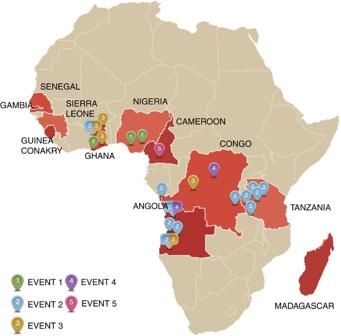Furthermore, sequence similarity searches (BLAST) of the genome of the South American oil palm, E. oleifera [3] , which does not produce the deep-violet coloured fruits similar to wild-type E. guineensis , do not identify an intact VIR gene. Figure 3: Geographic sources ofVIRmutant alleles. Palms were genotyped by sequencing to identify homozygosity or heterozygosity for each of the five identifiedVIRmutations (events 1–5). The location(s) of palms harbouring each of the mutation events in Africa is shown. Figure 3: Geographic sources of VIR mutant alleles. Palms were genotyped by sequencing to identify homozygosity or heterozygosity for each of the five identified VIR mutations (events 1–5). The location(s) of palms harbouring each of the mutation events in Africa is shown. Full size image Phylogeny, expression and function of VIR The R2R3-MYB family includes >100 genes in Arabidopsis [14] , [15] and >80 genes in maize [16] . The family includes two sets of imperfect repeats (R2 and R3), each including three alpha-helices forming a helix-turn-helix motif [17] . The R2R3 proteins are members of regulatory networks controlling development, metabolism and responses to biotic and abiotic stresses [18] . Phylogenetic analysis of the R2R3-MYB domain of VIR relative to MYB family members from various plant species indicates that VIR is most closely related to monocot Lilium LhMYB12 ( Fig. 4 ; Supplementary Figs 5 and 6 ). Although oil palm and Lilium are monocots, VIR and LhMYB12 cluster together within a distinct subgroup that is more similar to dicot cacao TcMYB113 and Arabidopsis PAP1, PAP2 and AtMYB113 than to monocot maize and rice C1. This classification is consistent with previous phylogenetic comparisons of LhMYB12, which place this MYB family protein in a subgroub with dicot MYB proteins including Arabidopsis PAP1 and PAP2, apple MYB10 and petunia AN2 and separate from a subgroup including monocot maize C1 (ref. 19 ). LhMYB12, PAP1 and AtMYB113 control accumulation of anthocyanins by regulation of expression of biosynthetic genes [20] , [21] , [22] . Expression levels of LhMYB12 are positively correlated with tepal anthocyanin pigmentation in Asiatic hybrid lilies [19] . Cacao TcMYB113 was recently identified as a likely candidate for regulation of green/red pod colour [23] . Overexpression of Arabidopsis PAP1 results in intense purple pigmentation in many vegetative organs throughout development, and ectopic expression in tobacco results in purple-pigmented plants [21] . Overexpression of AtMYB113 in Arabidopsis results in elevated pigment production, and downregulation of AtMYB113 , AtMYB114 , PAP1 and PAP2 results in anthocyanin deficiency [22] . Furthermore, overexpression of Arabidopsis Myb114 lacking the transactivation domain results in dominant anthocyanin deficiency [22] . The phylogenetic placement of VIR and LhMYB112 within a clade including mostly dicot MYB family proteins suggests that these MYB proteins represent a class of pigment-related regulators for which there are no extant orthologues in model monocots such as corn and rice. Although VIR is a member of a different clade of MYB proteins than maize C1, all five VIR mutations are intriguingly similar to McClintock’s maize C1-I allele in which a frameshift mutation in the carboxy-terminal region of C1 generates a dominant-negative protein resulting in reduced pigmentation [24] . Further, the last 20 amino acids of the oil palm protein are conserved in Lilium , but deleted from all 5 dominant alleles of VIR. These 20 amino acids share similarity with the C-terminal domain of C1 ( Supplementary Fig. 6 ). 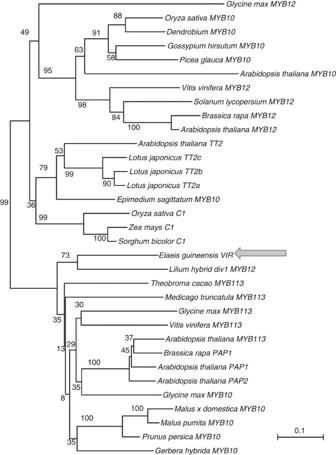These findings suggest that similar C-terminal truncation mechanisms result in anthocyanin deficiencies in oil palm. Figure 4: Phylogenetic analysis of VIR and various R2R3-MYB family members. Node numbers represent percentage of bootstrap replicates containing each clade. Placement of theElaeis guineensis VIRgene is designated by the arrow. Scale represents number of amino-acid changes per position within the alignment. Figure 4: Phylogenetic analysis of VIR and various R2R3-MYB family members. Node numbers represent percentage of bootstrap replicates containing each clade. Placement of the Elaeis guineensis VIR gene is designated by the arrow. Scale represents number of amino-acid changes per position within the alignment. Full size image In order to examine anthocyanin deficiency in virescens fruits, we performed a combination of metabolic and gene expression analyses. Spectrophotometric and chromatographic (high-performance liquid chromatography (HPLC)) analyses of acidified methanol extracts of exocarp confirmed the presence of anthocyanins in nigrescens , but absence in virescens fruit ( Fig. 5 ). Gene expression in nigresens and virescens whole fruits at 8 weeks after anthesis (WAA) was analysed by transcriptome sequencing ( Fig. 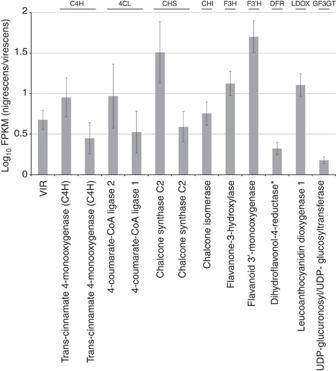Figure 6: Transcriptome analyses ofnigrescensandvirescenswhole fruit at 8 WAA. The average expression measured as fragments per thousand mapped reads (FPKM) for significantly (P<0.05, Student’st-test, two tailed, assuming equal variance) differentially expressed transcript reads matching genes in the rice anthocyanin phenylpropanoid pathway was calculated, and log10values of averagenigrescens/virescensare plotted with s.d. indicated by error bars. Gene groups are plotted in pathway order, suggesting thatvirescensfruits display impaired Myb/bHLH/WD-repeat-regulated gene expression beginning at the C4H step and extending through the anthocyanin pathway. Transcripts from four independent genes, two with homology to C4H and two with homology to C2, were coordinately regulated. *Annotation of transcripts by comparison with the rice proteome did not reveal transcripts annotated as dihydroflavonol reductase (DFR). However, a differentially expressed transcript has closest homology to the grapeDFRgene and is highly homologous toBrachypodiumandMedicagoDFR. 6 ; Supplementary Table 6 and Methods). The oil palm fruit typically exhibits biphasic growth with an initial growth spurt between ~4 and 9 WAA. Further, significant biochemical changes are observed starting at 8 WAA and up to 10 WAA during the transition phase between a metabolic sink and a storage sink [25] . Therefore, 8 WAA was chosen to examine expression of anthocyanin biosynthetic genes, avoiding later stages when expression of other mesocarp genes occurs that share the phenylpropanoid pathway, such as those involved in polyphenol biosynthesis. Transcriptome reads were annotated based on sequence comparisons with the rice proteome where possible. Transcriptome reads with substantial sequence similarity to biosynthetic genes in the anthocyanin phenylpropanoid pathway were identified ( Supplementary Table 7 ). Gene annotations are based solely on cross-species sequence comparisons and represent putative orthologues of anthocyanin pathway genes. Arabidopsis flavonoid enzymes can be divided into ‘early’ and ‘late’ groups that regulate distinct temporal stages of the pathway [26] . Late genes initiate at the dihydroflavonol reductase step, with downstream genes being regulated by Myb/bHLH/WD-repeat proteins [22] . However, in maize there is no early/late split [27] . At 8 WAA, nigrescens fruits display higher expression of VIR, as well as anthocyanin pathway genes starting at the trans-cinnamate 4-monooxygenase (C4H) step and extending throughout the anthocyanin biosynthetic pathway ( Fig. 6 ; Supplementary Fig. 7 ; Supplementary Table 7 ). These results suggest that the truncating VIR mutations result in coordinated dominant inhibition of MYB-regulated target gene expression at all steps of the anthocyanin pathway. Figure 5: Anthocyanin profiles in the virescens and nigrescens exocarp. ( a ) Exocarp extracts in acidic and alkaline conditions. The nigrescens extract was brilliant red in acidic conditions and turned green under alkaline conditions. The virescens extract, however, was light orange and did not change under alkaline conditions. ( b ) Ultraviolet–visible spectrophotometric profile of the extracts at pH 1.0. Nigrescens exhibited a maximum absorbance peak at about 520 nm. This peak was not observed in virescens . Anthocyanins are known to absorb strongly around this wavelength. ( c ) HPLC profile at 520 nm. The nigrescens extract had at least three major anthocyanin peaks at 520 nm, which were absent in virescens. Full size image Figure 6: Transcriptome analyses of nigrescens and virescens whole fruit at 8 WAA. The average expression measured as fragments per thousand mapped reads (FPKM) for significantly ( P <0.05, Student’s t -test, two tailed, assuming equal variance) differentially expressed transcript reads matching genes in the rice anthocyanin phenylpropanoid pathway was calculated, and log 10 values of average nigrescens/virescens are plotted with s.d. indicated by error bars. Gene groups are plotted in pathway order, suggesting that virescens fruits display impaired Myb/bHLH/WD-repeat-regulated gene expression beginning at the C4H step and extending through the anthocyanin pathway. Transcripts from four independent genes, two with homology to C4H and two with homology to C2, were coordinately regulated. *Annotation of transcripts by comparison with the rice proteome did not reveal transcripts annotated as dihydroflavonol reductase (DFR). However, a differentially expressed transcript has closest homology to the grape DFR gene and is highly homologous to Brachypodium and Medicago DFR. Full size image Our findings establish that the oil palm VIR gene controls fruit colour and that any one of five independent, but closely related, dominant mutations in the gene can cause the virescens fruit colour phenotype. Further demonstration of the effect of the VIR truncation mutations by transgenic approaches in model organisms, as well as the possible contributions of additional unidentified genetic variants to fruit colour phenotype are areas for future research. However, the discovery of the genetic basis of the role of VIR in the virescens phenotype paves the way for development of genetic testing for fruit colour well before planting and for the introgression of the desirable trait into elite breeding materials. For example, the identification of the VIR gene allows differentiation of the homozygous and heterozygous forms of virescens palms, as early as the seedling stage, and together with the recent identification of SHELL [4] , allows breeders to develop paternal ( pisifera ) lines that are homozygous for virescens for use in breeding programmes or for commercial seed production. All five alleles of VIR from equatorial Africa have mutations resulting in premature C-terminal truncations of the VIR protein, and their prevalence is unprecedented. This likely reflects dominant-negative inheritance (which makes novel alleles conspicuous) and cultural practices that retain the alleles for ritual purposes. The utility of these alleles will have important impacts on fruit harvesting practices, to improve oil yields and lead to improved land utilization. Plant materials and germplasm collection The mapping family used was derived from the self-pollination of a high-iodine value virescens tenera palm T128 (accession number MPOB 371), which has been described in detail [4] . An additional 108 palms derived from six families of different genetic backgrounds ( Supplementary Table 1 ) were available, part of which (81 palms) were used to confirm marker–trait association, while 96 of these palms were used to sequence the entire virescens gene. Similarly, an additional collection of advanced breeding lines (AVROS) (43 nigrecens ) and germplasm material (87 virescens and 353 nigrescens ) collected from seven countries in Africa were also sequenced to confirm the identity of the virescens gene and identify additional mutations within VIR . All germplasm materials were collected under bilateral agreements with the respective countries and followed closely the Convention on Biological Diversity (1992). Unopened leaf samples (spear leaves) were collected from individual palms and immediately frozen under liquid nitrogen and then stored at –80 °C until DNA preparation. DNA was extracted and purified from the leaf samples using the modified CTAB method [28] . Genetic mapping A total of 240 palms of the mapping family were available for DNA extraction at the start of this study. Of these, 32 palms could not be phenotyped with confidence, as the palms had been cut down or succumbed to disease before the fruit exocarp colour could be determined or re-confirmed. Of the 208 palms that were successfully phenotyped, 160 were identified as virescens palms and 48 as nigrescens palms. However, all 240 available palms were genotyped with 4,451 SNP markers using the Illumina iSelect assay (Illumina), 3 RFLP and 197 SSR markers. The genotype data were formatted for mapping according to an F 2 population. Markers showing segregation profile of 1:2:1 were used in the map construction. Two sets of genotype data were created, in which one was the converse of the other to account for phase differences in the T128 ‘selfed’ F 2 population. The genetic map was then constructed using JoinMap 4.0. Markers that exhibited severe distortion ( P <0.0001) and markers having >10% missing data were excluded. Both sets of genotype data were grouped at a recombination frequency of <0.2. Markers exhibiting nearest neighbour stress value >2 (cM) were identified and excluded from the analysis. Markers contributing to insufficient linkages were also removed. The T128 co-dominant map constructed comprised 16 groups, and VIR was placed on linkage group 1. Fruit colour phenotyping The fruit exocarp colour was determined on ripe bunches having at least one loose fruit per bunch (irrespective of plant height). The bunch was harvested from the tree and a minimum of five fruitlets was stripped from the bunch. Visual observation was made of the exocarp, and fruits were classified as nigrescens (reddish to deep violet) or virescens (orange) as seen from the apex [29] . In this study, at least two independent attempts were made to determine fruit colour of the mapping family as well as the breeding populations. With respect to the germplasm collection, fruit colour observations were made only once. Genome and transcriptome sequencing Twelve independent T128 progeny palms (five nigrescens and seven virescens ) were sequenced to × 20 raw sequence coverage by HISEQ 2000 (Illumina). For transcriptome sequencing, RNA was extracted from 10 to 20 fruits from 2 trees (1 nigrescens and 1 virescens ) at 8 WAA. Three replicate RNA extractions were performed for each fruit pool. TrueSeq (Illumina) libraries were constructed and sequenced by HISEQ 2000, generating 1/8 lane of reads per phenotype replicate. VIR Sanger sequencing The entirety of the VIR gene was amplified by PCR from oil palm genomic DNA using a forward primer sequence, 5′-GCGTACGTGGAACCACAA-3′, and reverse primer sequence, 5′-CTCCATTCTGGTGAGAAAGCGT-3′, generating a single ~2.9-kb amplicon. Forward and reverse primers included M13 Forward or M13 Reverse sequence tags, respectively. Amplicons were treated with exonuclease 1 (New England Biolabs) and shrimp alkaline phosphatase (Affymetrix) under standard conditions. Amplicons were sequenced using a combination of M13 primers and internal primers (internal primer sequences available upon request). Sequencing was performed on an ABI 3730 capillary DNA sequencer using big dye terminator VS 3.1 chemistry (Life Technologies). Local assemblies of each amplicon were constructed with PHRAP and reviewed in CONSED. Consensus sequence for each palm was aligned to the reference pisifera genome sequence [3] . Data were analysed to determine the integrity of the coding sequence and resulting putative translated polypeptide for each palm. A large percentage of the palms analysed were part of the 110,000 diverse germplasm collection available at MPOB. Phylogenetic analysis A collection of R2R3 MYBs from previously studied plant species were selected based on their similarity to the VIR protein. These sequences were aligned using the ClustalX program, and the highly conserved R2R3 domains were then processed using the Neighbor Joining method with 1,000 bootstrap replicates [30] . Pigment extraction Acidified methanol (1% HCl, v/v) was added to ground exocarp slices of E. guineensis (15WAA nigrescens and virescens fruits) and stirred to ensure efficient extraction of pigments. The extracts were centrifuged at 3,000 g in an Eppendorf 5810R centrifuge to remove debris. The supernatants were removed and filtered before further analysis. Spectrophotometric and chromatographic analyses were carried out to determine the presence, if any, of anthocyanins. Equal weights of E. guineensis virescens and nigrescens exocarp materials were used for extraction under identical conditions. Spectrophotometry Ultraviolet–visible absorption spectra were recorded from 230 to 780 nm at 10 nm intervals using a U-2800 double beam scanning ultraviolet–visible spectrophotometer (Hitachi, Japan). HPLC HPLC was performed on a Waters 250 × 4.6 mm i.d., 5 μm, Atlantis dC18 column using a Waters Alliance W 2695 Separation Module (Waters Assoc., Milford, USA) equipped with a 2996 photodiode array detector. A gradient mobile phase comprising solvent (A)—9% acetonitrile, 10% formic acid, 81% water (v/v/v) and solvent (B)—36% acetonitrile, 10% formic acid, 54% water (v/v/v) was used. The elution gradient was 0–3 min, 100% A, 3–30 min 71.5% A, 28.5% Band 30–45 min, 71.5% A, 28.5% B. The flow rate was 1.0 ml min −1 and injection volume was 20 μl. Absorbance spectra were collected for all peaks. Transcriptome analysis Whole-transcriptome sequencing analysis was performed on each of three replicates for pools of 10–20 fruits of nigrescens or virescens phenotypes (Illumina). Transcripts were mapped and identified based on similarity to the rice proteome where possible. One pathway step (dihydroflavonol reductase) not identified by similarity to the rice proteome was annotated by comparison of translated sequence with all non-redundant peptide databases. Measurements of zero fragments per 1,000 mapped reads (FPKM) were not included in calculating the mean and s.d., and only transcripts with FPKM values greater than zero in at least two of three replicates per phenotype were included. Ratios for all pairwise comparisons of nigrescens versus virescens replicates were averaged and plotted as log 10 ( nigrescens FPKM /virescens FPKM). How to cite this article: Singh, R. et al . The oil palm VIRESCENS gene controls fruit colour and encodes a R2R3-MYB. Nat. Commun. 5:4106 doi: 10.1038/ncomms5106 (2014). Accession codes: Transcriptome data has been deposited in GenBank/EMBL/DDBJ sequence read archive (SRA) under the accession code SUB497076 . Annotated genomic sequence of the VIR gene from the reference E. guineensis genome has been deposited in GenBank/EMBL/DDBJ nucleotide core database under the accession code KJ789862 .